Switching between humoral and cellular immune responses inDrosophilais guided by the cytokine GBP Insects combat infection through carefully measured cellular (for example, phagocytosis) and humoral (for example, secretion of antimicrobial peptides (AMPs)) innate immune responses. Little is known concerning how these different defense mechanisms are coordinated. Here, we use insect plasmatocytes and hemocyte-like Drosophila S2 cells to characterize mechanisms of immunity that operate in the haemocoel. We demonstrate that a Drosophila cytokine, growth-blocking peptides (GBP), acts through the phospholipase C (PLC)/Ca 2+ signalling cascade to mediate the secretion of Pvf, a ligand for platelet-derived growth factor- and vascular endothelial growth factor-receptor (Pvr) homologue. Activated Pvr recruits extracellular signal-regulated protein kinase to inhibit humoral immune responses, while stimulating cell ‘spreading’, an initiating event in cellular immunity. The double-stranded RNA (dsRNA)-targeted knockdown of either Pvf2 or Pvr inhibits GBP-mediated cell spreading and activates AMP expression. Conversely, Pvf2 overexpression enhances cell spreading but inhibits AMP expression. Thus, we describe mechanisms to initiate immune programs that are either humoral or cellular in nature, but not both; such immunophysiological polarization may minimize homeostatic imbalance during infection. Many components of innate immunity share an ancient origin in metazoan evolution, and so Drosophila has long been considered as a relevant and genetically tractable model for studying general mechanisms of innate immunity in animals [1] . For example, in Drosophila larvae, the major blood immunoreactive cells that defend the haemocoel against its invasion by foreign organisms are plasmatocytes [1] , [2] , [3] , which normally comprise 90–95% of all mature hemocytes [4] , [5] , [6] . Plasmatocytes, which exhibit both cellular and humoral immune activities, are considered to be equivalent to mammalian cells of the monocyte/macrophage lineage [7] . The main cellular responses of plasmatocytes are phagocytosis and encapsulation; humoral responses involve the synthesis and secretion of antimicrobial peptides (AMPs). More recent studies have revealed that changes in innate immune activities can also combat non-infectious stresses and participate in maintenance of organismic homeostasis [8] , [9] . Ideally, there should be minimal disturbance of these homeostatic functions, and thus protection from collateral tissue damage, when immune cells are mobilized against invading pathogens [9] , [10] . Thus the processes of immunity and inflammation are anticipated to involve careful coordination and intricate cross-talk between multiple stimulatory as well as inhibitory signalling pathways, but the mechanisms are poorly understood. In a variety of insect species, cytokine-mediated activation of plasmatocyte cell spreading is a prelude to these cells becoming competent to perform phagocytosis and encapsulation (that is, the process of cellular immunity) [2] , [11] . Many of these cytokines, which have variously been described as either growth-blocking peptides (‘GBPs’) [8] , or plasmatocyte-spreading peptides [8] , [12] , [13] , [14] , are activated on their release from the C terminus of larger propeptides by serine protease activity. These bioactive peptides contain a consensus motif: Cx 2 Gx (4–6) Gx (1−2) C[K/R] [13] . The active form of Drosophila GBP contains 24 amino-acid residues; overexpression of GBP in Drosophila larvae increases the expression of antimicrobial peptide (AMP) genes such as Metchnikowin ( Mtk ) and Diptericin ( Dpt ), which are markers for humoral aspects of innate immunity [8] . In Drosophila , GBP also regulates immune responses to non-infectious environmental challenges such as physical stress or exposure to temperature changes [8] . The current study investigates both positive and negative cell-signalling control over immune responses to Drosophila GBP. However, plasmatocytes are not an ideal model system for studying immune responses, because their isolation is a tedious procedure, which yields only limited quantities of cells. Thus, another goal in our study is to develop a more tractable cell model to study GBP-dependent immunological mechanisms. Previous work has shown that Drosophila S2 cells recapitulate key elements of the innate immune program [15] , [16] , [17] . S2 cells are derived from embryonic hemocyte lineages, and they are able to phagocytose microbes and secrete AMP [7] . The experiments described in this study lead us to uncover a linear pathway by which GBP is as an upstream activator of the platelet-derived growth factor- and vascular endothelial growth factor-receptor homologue (Pvr). The latter finding was initially unexpected as previous work has indicated that Pvr enforces an inhibitory pathway in humoral innate immunity [18] . Indeed, in the current study, we confirm that activation of Pvr downstream of GBP restrains expression of AMPs in both plasmatocytes and S2 cells. However, we also demonstrate that the Pvr cascade activates cellular aspects of the innate immune pathway. That is, the innate immune functionality of plasmatocytes per se is not inhibited by Pvr, but rather, the nature of their immune response is reprogrammed. In this way, we demonstrate that individual cells respond to the different roles of GBP by becoming polarized to exhibit either the humoral or cellular arm of the innate immune process. Cell spreading in Pseudaletia separata and Drosophila plasmatocytes Cytokine-induced cell spreading offers a phenotypic readout of the first step in the activation of the cellular arm of the innate immune pathway. Plasmatocyte spreading is characterized by an increased adhesion to foreign surfaces and a change from a spherical shape into a more flattened and extended morphology that can be readily quantified [12] , [14] . P. separata GBP (PsGBP) [19] , [20] , [21] and Drosophila GBP [8] induced these morphological changes in plasmatocytes isolated from larvae of the armyworm P. separata ( Fig. 1a ) and Drosophila ( Fig. 1b ), respectively. As in previous studies, we employed the active version of these peptides that are released following serine protease action on the inactive propeptide precursors [8] , [13] . 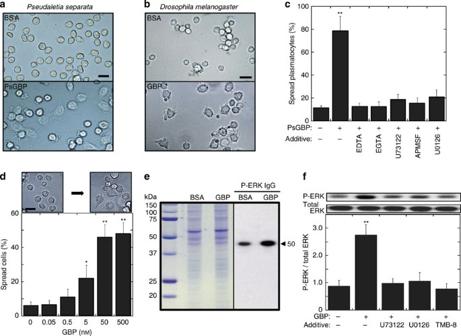Figure 1: Spreading response of plasmatocytes andDrosophilaS2 cells. (a) Representative images ofP. separatelarval plasmatocytes incubated with either 20 nM PsGBP (lower) or BSA (upper) for 30 min. Scale bar, 25 μm. (b) Representative images ofDrosophilalarval plasmatocytes incubated with either 20 nM GBP (lower) or BSA (upper) for 20 min. Scale bar, 20 μm. (c) Quantification of PsGBP-mediated spreading activity ofP. separatelarval plasmatocytes. Where indicated, either 10 mM EDTA, 10 mM EGTA, 10 μM U73122, 100 μM APMSF or 10 μM U0126 was added 5 min before 20 nM PsGBP. Each bar represents the mean±s.d. for eight independent determinations. **P<0.01: Significant differences from control (−GBP/−Additive) value are indicated by Tukey’s HSD. (d) Representative images (upper) of 50 nM GBP-induced spreading of S2 cells and quantification of cell spreading (lower) 30 min after addition of the indicated concentration of GBP. Each value represents the mean±s.d. for six independent determinations *P<0.05; **P<0.01: Significant differences from control (0 nM GBP) value are indicated by Tukey’s HSD. Scale bar, 20 μm. (e) Western blots of GBP-induced phosphorylation of ERK in S2 cells. Coomassie Brilliant Blue stained SDS/PAGE gel (left), and immunoblotting with phosphorylated ERK IgG (right). The arrowhead indicates the ERK band. (f) The inhibition of GBP-induced ERK activation. Where indicated, either 10 μM U73122, 10 μM U0126, or 10 μM TMB-8 was added 10 min before 20 nM GBP and ERK was assayed after 3 min-incubation with GBP. Each bar represents the mean±s.d. for four independent determinations. **P<0.01: Significantly different from control (−GBP/-Additive) value. Full blot is supplied inSupplementary Fig. 10. Figure 1: Spreading response of plasmatocytes and Drosophila S2 cells. ( a ) Representative images of P. separate larval plasmatocytes incubated with either 20 nM PsGBP (lower) or BSA (upper) for 30 min. Scale bar, 25 μm. ( b ) Representative images of Drosophila larval plasmatocytes incubated with either 20 nM GBP (lower) or BSA (upper) for 20 min. Scale bar, 20 μm. ( c ) Quantification of PsGBP-mediated spreading activity of P. separate larval plasmatocytes. Where indicated, either 10 mM EDTA, 10 mM EGTA, 10 μM U73122, 100 μM APMSF or 10 μM U0126 was added 5 min before 20 nM PsGBP. Each bar represents the mean±s.d. for eight independent determinations. ** P <0.01: Significant differences from control (−GBP/−Additive) value are indicated by Tukey’s HSD. ( d ) Representative images (upper) of 50 nM GBP-induced spreading of S2 cells and quantification of cell spreading (lower) 30 min after addition of the indicated concentration of GBP. Each value represents the mean±s.d. for six independent determinations * P <0.05; ** P <0.01: Significant differences from control (0 nM GBP) value are indicated by Tukey’s HSD. Scale bar, 20 μm. ( e ) Western blots of GBP-induced phosphorylation of ERK in S2 cells. Coomassie Brilliant Blue stained SDS/PAGE gel (left), and immunoblotting with phosphorylated ERK IgG (right). The arrowhead indicates the ERK band. ( f ) The inhibition of GBP-induced ERK activation. Where indicated, either 10 μM U73122, 10 μM U0126, or 10 μM TMB-8 was added 10 min before 20 nM GBP and ERK was assayed after 3 min-incubation with GBP. Each bar represents the mean±s.d. for four independent determinations. ** P <0.01: Significantly different from control (−GBP/-Additive) value. Full blot is supplied in Supplementary Fig. 10 . Full size image Previous work has shown that extracellular Ca 2+ is required in order that hemocyte spreading can be induced by plasmatocyte-spreading peptides from Spodoptera exigua [22] . Likewise, we also found that PsGBP-dependent spreading of P. separata plasmatocytes was inhibited when extracellular Ca 2+ was chelated with either EDTA or EGTA ( Fig. 1c ). Recently, we demonstrated that extracellular Ca 2+ is also required for maximizing the intracellular Ca 2+ signal that GBP elicits from Drosophila S3 cells on its activation of PLC [23] . We therefore investigated if this signalling response might participate in plasmatocyte spreading. Inhibition of PLC in P. separata plasmatocytes by addition of U73122 prevented PsGBP from inducing cell spreading ( Fig. 1c ). Furthermore, we also made the novel observation that PsGBP-dependent activation of plasmatocytes was attenuated by (p-amidinophenyl)methylsulphonyl fluoride (APMSF), a serine protease inhibitor ( Fig. 1c ). Since active PsGBP was used in these assays, the inhibition by APMSF suggested that the processing of a different precursor protein might be involved in PsGBP-induced spreading of plasmatocytes. Cellular activation of S2 cells by GBP The isolation of plasmatocytes from Drosophila larvae is a tedious procedure that yields relatively few cells. One of the goals of our study was to develop a more tractable cell model system in which to study the GBP-dependent signalling mechanisms that promote plasmatocyte spreading in Drosophila [16] , [17] . It is known that S2 cells are likely derived from embryonic hemocyte lineages [7] . In addition, we have noted that S2 cells incubated for extended periods in a microplate slowly develop a plasmatocyte-like ‘spreading’ phenotype and also encapsulate foreign objects such as dextran beads ( Supplementary Fig. 1a,b ). We have now made the notable observation that Drosophila GBP significantly accelerated the acquisition of the spreading phenotype in a concentration-dependent manner ( Fig. 1d , Supplementary Fig. 1b ). These observations led us to use S2 cells as a model for characterizing the GBP-induced signalling events that promote cell spreading. Extracellular signal-regulated protein kinase activation by GBP In earlier work with the MaBr4 fat body cell line from Lepidoptera Mamesta brassicae , we found that M. brassicae GBP activates the extracellular signal-regulated protein kinase (ERK) [24] . Western blotting revealed that GBP stimulated phosphorylation of Drosophila ERK (the gene product of rolled ) in S2 cells ( Fig. 1e ). We next found that GBP-induced ERK activation was blocked by the addition of either a PLC inhibitor (U73122) or an inositol triphosphate (IP 3 ) receptor (Itpr) antagonist (TMB-8) ( Fig. 1f ). These data indicate that ERK lies downstream of PLC activation. We confirmed that Drosophila GBP activated PLC in S2 cells by high-performance liquid chromatography (HPLC) analysis of inositol phosphate levels in control and GBP-stimulated S2 cells ( Fig. 2a ). We further found that GBP elevated levels of 1,4,5 IP 3 and 1,4,5,6 IP 4 4-5 fold ( Fig. 2b ). The former promotes calcium mobilization [25] , and the latter is a transcriptional regulator [26] . 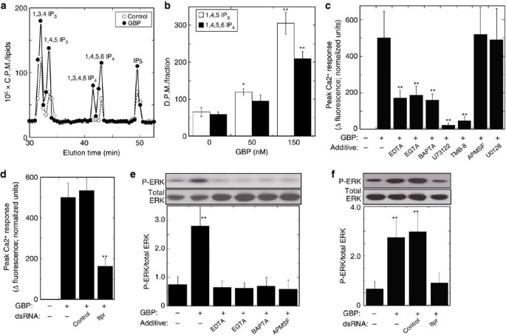Figure 2: Characterization of GBP-dependent signalling inDrosophilaS2 cells. (a) Q-100 SAX HPLC analysis of the [3H]-labelled inositol phosphates in S2 cells treated with either 50 nM GBP or vehicle for 45 min. [3H]-labelled inositol phosphates were analysed using a 4.6 × 250 mm Q-100 HPLC column (Thomson Instruments, USA) with an in-line detector. (b) Effects of GBP on the level of 1,4,5 IP3and 1,4,5,6 IP4. Each value represents the mean±s.d. for three independent determinations *P<0.05; **P<0.01: Significant differences from control (0 nM GBP) value are indicated by Tukey’s HSD. (c) Characterization of the nature of GBP-induced intracellular Ca2+elevation in GCaMP3-expressing S2 cells. Where indicated, either 10 mM EDTA, 10 mM EGTA, 10 mM BAPTA, 10 μM U73122, 10 μM TMB-8, 100 μM APMSF or 10 μM U0126 was added 10 min before 20 nM GBP. Peak Ca2+-dependent fluorescence signals were normalized to control (+GBP/–Additive) values to indicate relative maximum Ca2+signals. Each value represents the mean±s.d. for three independent determinations. **P<0.01: Significant differences from control (+GBP/–Additive) value are indicated by Tukey’s HSD. (d) The inhibition of GBP-induced intracellular Ca2+elevation in GCaMP3-expressing S2 cells by dsRNA targeting ofItpr. A 500 bp irrelevant dsRNA from the MEGAscriptTMdsRNA Kit (Life Technologies, USA) served as a negative control. **P<0.01: Significant difference from control (+GBP/–dsRNA) value is indicated by Tukey’s HSD. Other explanations are as in (c). (e) Effects on 3 min of GBP-induced activation of ERK in S2 cells when either calcium chelators (10 mM EDTA, 10 mM EGTA, 10 mM BAPTA) or serine protease inhibitor (100 μM APMSF) was added 10 min before 20 nM GBP. Each value represents the mean±s.d. for five independent determinations. **P<0.01: Significant difference from control (−GBP/–Additive) value is indicated by Tukey’s HSD. Full blot was supplied inSupplementary Fig. 10. (f) Effects of dsRNA targeting ofItpron GBP-dependent activation of ERK. **P<0.01: Significant differences from control (–GBP/–dsRNA) value are indicated by Tukey’s HSD. Other explanations are as ind. Full blot is supplied inSupplementary Fig. 10. Figure 2: Characterization of GBP-dependent signalling in Drosophila S2 cells. ( a ) Q-100 SAX HPLC analysis of the [ 3 H]-labelled inositol phosphates in S2 cells treated with either 50 nM GBP or vehicle for 45 min. [ 3 H]-labelled inositol phosphates were analysed using a 4.6 × 250 mm Q-100 HPLC column (Thomson Instruments, USA) with an in-line detector. ( b ) Effects of GBP on the level of 1,4,5 IP 3 and 1,4,5,6 IP 4 . Each value represents the mean±s.d. for three independent determinations * P <0.05; ** P <0.01: Significant differences from control (0 nM GBP) value are indicated by Tukey’s HSD. ( c ) Characterization of the nature of GBP-induced intracellular Ca 2+ elevation in GCaMP3-expressing S2 cells. Where indicated, either 10 mM EDTA, 10 mM EGTA, 10 mM BAPTA, 10 μM U73122, 10 μM TMB-8, 100 μM APMSF or 10 μM U0126 was added 10 min before 20 nM GBP. Peak Ca 2+ -dependent fluorescence signals were normalized to control (+GBP/–Additive) values to indicate relative maximum Ca 2+ signals. Each value represents the mean±s.d. for three independent determinations. ** P <0.01: Significant differences from control (+GBP/–Additive) value are indicated by Tukey’s HSD. ( d ) The inhibition of GBP-induced intracellular Ca 2+ elevation in GCaMP3-expressing S2 cells by dsRNA targeting of Itpr . A 500 bp irrelevant dsRNA from the MEGAscript TM dsRNA Kit (Life Technologies, USA) served as a negative control. ** P <0.01: Significant difference from control (+GBP/–dsRNA) value is indicated by Tukey’s HSD. Other explanations are as in ( c ). ( e ) Effects on 3 min of GBP-induced activation of ERK in S2 cells when either calcium chelators (10 mM EDTA, 10 mM EGTA, 10 mM BAPTA) or serine protease inhibitor (100 μM APMSF) was added 10 min before 20 nM GBP. Each value represents the mean±s.d. for five independent determinations. ** P <0.01: Significant difference from control (−GBP/–Additive) value is indicated by Tukey’s HSD. Full blot was supplied in Supplementary Fig. 10 . ( f ) Effects of dsRNA targeting of Itpr on GBP-dependent activation of ERK. ** P <0.01: Significant differences from control (–GBP/–dsRNA) value are indicated by Tukey’s HSD. Other explanations are as in d . Full blot is supplied in Supplementary Fig. 10 . Full size image We demonstrated that GBP significantly elevated intracellular Ca 2+ concentrations in S2 cells in a concentration-dependent manner ( Supplementary Fig. 2a,b ). The GBP-induced elevation of Ca 2+ concentration was significantly repressed by the chelation of extracellular Ca 2+ by the addition of either EDTA, EGTA or BAPTA or by inhibition of PLC by U73122 ( Fig. 2c ). We furthermore confirmed the contribution of the PLC/IP 3 cascade by showing that GBP-dependent Ca 2+ elevation was inhibited by dsRNA-mediated knockdown of Itpr expression in S2 cells ( Fig. 2d ) as well as the Itpr antagonist (TMB-8) ( Fig. 2c ). Chelation of extracellular Ca 2+ by the addition of EDTA, EGTA or BAPTA substantially reduced GBP-induced activation of ERK ( Fig. 2e ). Moreover, cell treatment with dsRNA against Itpr also repressed GBP-dependent ERK activation ( Fig. 2f ) and cell spreading in S2 cells ( Supplementary Fig. 3 ). Thus, PLC activation by GBP has immunophysiological consequences. Furthermore, we found that the MEK inhibitor U0126 did not affect GBP-induced elevation of intracellular Ca 2+ ( Fig. 2c ), consistent with ERK activation lying downstream of intracellular Ca 2+ elevation. There are several intracellular signalling pathways that directly couple Ca 2+ mobilization to ERK activation [27] , [28] . However, this does not seem to be the case in our experiments, because the stimulation of ERK phosphorylation by GBP was inhibited by the serine protease inhibitor APMSF ( Fig. 2e ). Since APMSF did not affect the ability of GBP to mobilize Ca 2+ ( Fig. 2c ), and in any case the bioactive form of GBP was used, these results indicate that GBP-mediated activation of ERK involves protease-dependent signalling events that are downstream of Ca 2+ mobilization. Therefore, we next sought further information concerning the mechanisms that are involved. GBP-induced signalling events lead to Pvr activation Previous reports have shown that ERK can be activated by the Pvf/Pvr signalling pathway in hemocytes of Drosophila larvae and embryos [29] , [30] . Furthermore, Pvr ligands (Pvfs) and Pvr have been reported to act upstream of Ras/MAPK in S2 cells [31] . However, it has not previously been considered that GBP might activate Pvf/Pvr signalling; therefore, we next examined that very possibility. The Drosophila genome encodes three forms of Pvf (types 1, 2 and 3) [29] . Real-time PCR (RT–PCR) analysis showed that Pvf2 is expressed at much higher levels than Pvf1 and Pvf3 in S2 cells ( Supplementary Fig. 4a ). We further found that knockdown of Pvf2 expression by RNA interference (RNAi) reduced GBP-induced activation of ERK ( Fig. 3a ). RNAi knockdown of Pvr also abolished GBP-dependent ERK activation ( Fig. 3a ). In contrast, knockdown of either Pvf1 or Pvf3 expression had no effects on ERK activation ( Fig. 3a ; Supplementary Fig. 4b ). These data reinforce the particular importance of Pvf2, although they do not exclude a redundant role for Pvf1 and Pvf3, for example in forming heterodimers with Pvf2. Furthermore, we took the conditioned medium that had been used to culture S2 cells in which Pvf2 was overexpressed (see Supplementary Fig. 5 ), and added that to naïve S2 cells; that procedure activated ERK while the activation was neutralized when the conditioned medium was preincubated with anti-Pvf2 IgG ( Fig. 3b ). These data not only indicate that Pvf2 was present in the conditioned medium, but also demonstrate that the Pvf2 was biologically active. By western blot analysis, we also demonstrated that Pvf2 concentrations were increased in culture medium of S2 cells following either the addition of GBP, or the addition of the Ca 2+ ionophore, A23187 ( Fig. 3c ). Liquid chromatography mass spectrometry analysis of the immunoreactive band confirmed the presence of Pvf2 ( Supplementary Fig. 6 ). Further evidence of the role of Ca 2+ was obtained by showing that the release of Pvf2 by GBP was inhibited when Ca 2+ mobilization was inhibited on the chelation of extracellular Ca 2+ by EGTA ( Fig. 3c ). In conclusion, we have demonstrated that GBP-mediated activation of ERK is dependent on Ca 2+ -dependent Pvf2 secretion into the culture medium, and the presence of the Pvr. 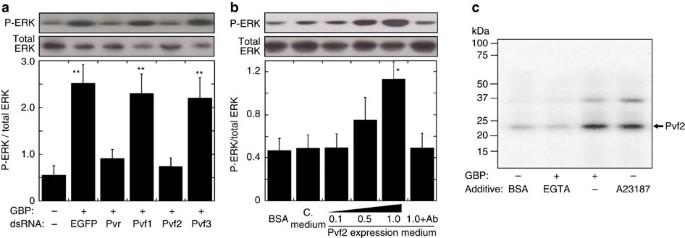Figure 3: Analysis of the Pvf/Pvr and ERK mediated cell spreading response inDrosophilaS2 cells. (a) Effects of dsRNA targeting of eitherPvrorPvf 1-3genes on GBP-dependent ERK activation in S2 cells. S2 cells were used three days after adding dsRNA of each target gene as described in the Methods. Where indicated, 20 nM GBP was added for 3 min. Each value represents the mean±s.d. for four independent determinations. **P<0.01: Significant differences from control (–GBP/–dsRNA) value are indicated by Tukey’s HSD. Full blot was supplied inSupplementary Fig. 11. (b) ERK activation by conditioned medium ofPvf2-over-expressing S2 cells. 0.1, 0.5, 1.0: 10-fold diluted, 2-fold diluted and undiluted conditioned media of S2 cell culture (5 × 106cells per well) were respectively used. C. medium: medium from cultures of control S2 cells. 1.0+Ab: undiluted conditioned medium preincubated with anti-Pvf2 antibody for 2 h. Each value represents the mean±s.d. for five independent determinations. *P<0.05: Significant difference from control (BSA) value is indicated by Tukey’s HSD. Full blot is supplied inSupplementary Fig. 11. (c) Western blot of Pvf2 protein in incubation medium of S2 cells stimulated by either 20 nM GBP or 100 nM A23187 for 3 min. In the case of EGTA treatment, S2 cells were preincubated with 10 mM EGTA for 10 min before addition of 20 nM GBP. Liquid chromatography mass spectrometry analysis of the immunoreactive band indicated by the arrow (in GBP-treated sample) showed that two determined peptide fragment sequences &#8232;(VPRPEVVHITR and PRPEVVHITR) were found to be completely identical in Pvf2 amino-acid sequence, indicating that this band is Pvf2 precursor protein (seeSupplementary Fig. 6). Figure 3: Analysis of the Pvf/Pvr and ERK mediated cell spreading response in Drosophila S2 cells. ( a ) Effects of dsRNA targeting of either Pvr or Pvf 1-3 genes on GBP-dependent ERK activation in S2 cells. S2 cells were used three days after adding dsRNA of each target gene as described in the Methods. Where indicated, 20 nM GBP was added for 3 min. Each value represents the mean±s.d. for four independent determinations. ** P <0.01: Significant differences from control (–GBP/–dsRNA) value are indicated by Tukey’s HSD. Full blot was supplied in Supplementary Fig. 11 . ( b ) ERK activation by conditioned medium of Pvf2 -over-expressing S2 cells. 0.1, 0.5, 1.0: 10-fold diluted, 2-fold diluted and undiluted conditioned media of S2 cell culture (5 × 10 6 cells per well) were respectively used. C. medium: medium from cultures of control S2 cells. 1.0+Ab: undiluted conditioned medium preincubated with anti-Pvf2 antibody for 2 h. Each value represents the mean±s.d. for five independent determinations. * P <0.05: Significant difference from control (BSA) value is indicated by Tukey’s HSD. Full blot is supplied in Supplementary Fig. 11 . ( c ) Western blot of Pvf2 protein in incubation medium of S2 cells stimulated by either 20 nM GBP or 100 nM A23187 for 3 min. In the case of EGTA treatment, S2 cells were preincubated with 10 mM EGTA for 10 min before addition of 20 nM GBP. Liquid chromatography mass spectrometry analysis of the immunoreactive band indicated by the arrow (in GBP-treated sample) showed that two determined peptide fragment sequences &#8232;(VPRPEVVHITR and PRPEVVHITR) were found to be completely identical in Pvf2 amino-acid sequence, indicating that this band is Pvf2 precursor protein (see Supplementary Fig. 6 ). Full size image Immunophysiological role of the Pvr–ERK signalling pathway We next found that the MEK inhibitor, U0126, significantly repressed activation of ERK, both in S2 cells treated with GBP ( Fig. 1f ), and in PsGBP-treated plasmatocytes prepared from the armyworm larvae ( Fig. 1c ). Furthermore, U0126 inhibited PsGBP-induced spreading of P. separata plasmatocytes ( Supplementary Fig. 7 ). These results together with the above observation that RNAi knockdown of Itpr repressed GBP-induced spreading as well as ERK activation in S2 cells ( Fig. 2f ; Supplementary Fig. 3 ) indicate the importance of ERK activation for cell spreading. Moreover, dsRNA targeting of either ERK, Pvr or Pvf2 significantly repressed the GBP-induced spreading in S2 cells ( Fig. 4a–c ). 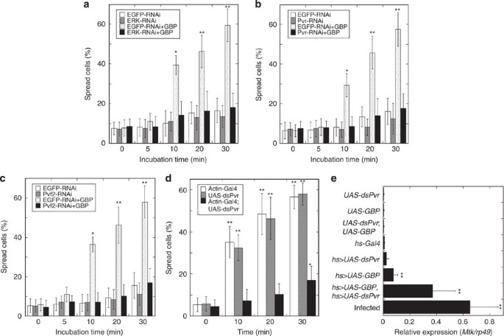Figure 4: Effects of altered expression of Pvf/Pvr–ERK signalling related genes on cell spreading andMetchnikowinexpression. (a–c) Effect of dsRNA targeting ofErk(a),Pvr(b), orPvf2(c) on spreading ofDrosophilaS2 cells stimulated by 50 nM GBP for the indicated times. Each value represents the mean±s.d. for 3–7 independent determinations. *P<0.05; **P<0.01: Significant differences from control (0 min, EGFP-RNAi) value are indicated by Tukey’s HSD. (d) Effect of dsRNA targeting ofPvron GBP-induced spreading of plasmatocytes ofDrosophilalarvae. Plasmatocytes prepared from test larvae were incubated with 20 nM GBP (see Materials and Methods). Average rates of spread plasmatocytes prepared from any test larvae were less than 20% when they were incubated with 20 nM BSA for 30 min. Each value represents the mean±s.d. for six independent determinations. *P<0.05; **P<0.01: Significant differences from control (0 min, Actin-Gal4) value are indicated by Tukey’s HSD. (e) Analysis of hemocyteMtkexpression withPvrknockdown backgrounds under forced expression ofGBPinDrosophilalarvae by quantitative real-time PCR. Thehs-Gal4-dependent knockdown ofPvrand overexpression ofGBPwere induced by heat treatment at 35 °C for 30 min twice with 12 h-interval. Infection was induced by stabbing third instar larvae with a thin tungsten needle previously dipped into a concentrated culture ofSerratia marcescens3 h before measuringMtkexpression. Induction ofMtkexpression by forcedGBPexpression was measured in larvae whosePvrexpression was significantly repressed as shown inSupplementary Fig. 8. Each value represents the mean±s.d. for five independent determinations. **P<0.01: Significant differences from control (UAS-dsPvr;UAS-GBP) value are indicated by Tukey’s HSD. Figure 4: Effects of altered expression of Pvf/Pvr–ERK signalling related genes on cell spreading and Metchnikowin expression. ( a – c ) Effect of dsRNA targeting of Erk ( a ), Pvr ( b ), or Pvf2 ( c ) on spreading of Drosophila S2 cells stimulated by 50 nM GBP for the indicated times. Each value represents the mean±s.d. for 3–7 independent determinations. * P <0.05; ** P <0.01: Significant differences from control (0 min, EGFP-RNAi) value are indicated by Tukey’s HSD. ( d ) Effect of dsRNA targeting of Pvr on GBP-induced spreading of plasmatocytes of Drosophila larvae. Plasmatocytes prepared from test larvae were incubated with 20 nM GBP (see Materials and Methods). Average rates of spread plasmatocytes prepared from any test larvae were less than 20% when they were incubated with 20 nM BSA for 30 min. Each value represents the mean±s.d. for six independent determinations. * P <0.05; ** P <0.01: Significant differences from control (0 min, Actin-Gal4) value are indicated by Tukey’s HSD. ( e ) Analysis of hemocyte Mtk expression with Pvr knockdown backgrounds under forced expression of GBP in Drosophila larvae by quantitative real-time PCR. The hs-Gal4 -dependent knockdown of Pvr and overexpression of GBP were induced by heat treatment at 35 °C for 30 min twice with 12 h-interval. Infection was induced by stabbing third instar larvae with a thin tungsten needle previously dipped into a concentrated culture of Serratia marcescens 3 h before measuring Mtk expression. Induction of Mtk expression by forced GBP expression was measured in larvae whose Pvr expression was significantly repressed as shown in Supplementary Fig. 8 . Each value represents the mean±s.d. for five independent determinations. ** P <0.01: Significant differences from control ( UAS-dsPvr ; UAS-GBP ) value are indicated by Tukey’s HSD. Full size image As mentioned above, cell spreading offers a phenotypic readout of the first step in the activation of the cellular arm of the innate immune pathway. Thus, our data demonstrated that GBP promotes cellular immune responses through the activation of the Pvf/Pvr–ERK signalling pathway. We reinforced this idea by demonstrating that plasmatocytes prepared from Drosophila larvae treated with Pvr dsRNA were significantly impaired in their capacity to acquire spread morphology on addition of GBP ( Fig. 4d ). That conclusion may at first sight appear to be inconsistent with previous report characterizing the Pvr pathway as inhibiting innate immunity [18] . However, the latter conclusion is based on the earlier demonstration that the Pvr cascade inhibits AMP synthesis [18] –a humoral response–whereas our experiments show that a separate, cellular arm of the innate immune program is activated. We therefore sought to clarify the effects of Pvr expression on the relationship between GBP-induced humoral and cellular immune responses using transgenic Drosophila larvae. We examined expression of Mtk in the hemocytes of Drosophila larvae in which GBP was overexpressed. In agreement with an earlier study [8] , we found that GBP slightly but significantly increased Mtk expression, but to a level that was about 10-fold below that seen in larvae after introducing S. marcescens in an acute model of septic injury ( Fig. 4e ). Moreover, an important new observation in the current study is that the GBP-induced Mtk expression level was enhanced almost fivefold in Pvr knockdown larvae ( Fig. 4e ; controls validating the expected changes in GBP and Pvr expression are shown in Supplementary Fig. 8 ). These data show that, in non-infected control larvae, it is the Pvf/Pvr signalling cascade that prevents GBP from maximally stimulating Mtk expression. Thus, when Pvr expression was knocked down, the GBP-mediated Mtk expression attained a level that was only 40% less than that observed in the septic injury model ( Fig. 4e ). We further showed that the GBP-dependent Mtk and Dpt expression levels were significantly enhanced in S2 cells treated with Pvf2 dsRNA compared with those in control S2 cells ( Fig. 5a,b ). That is, our data indicate that Pvf2 inhibits this humoral arm of the GBP-induced immune responses. We next examined the effects on cellular and humoral immune responses when Pvf2 was overexpressed under the control of the Cu 2+ -inducible metallothionein promoter ( Supplementary Fig. 5 ). We found that Pvf2 overexpression enhanced spreading of S2 cells irrespective of the presence of GBP ( Fig. 5c ). On the other hand, GBP-induced Mtk and Dpt expression levels were significantly repressed by overexpression of Pvf2 compared with control S2 cells ( Fig. 5d,e ). In conclusion, our data indicate that the Pvf2/Pvr signalling cascade polarizes the nature of the immune responses of S2 cells and plasmatocytes in favour of mediating the cellular arm of the innate immune pathway. 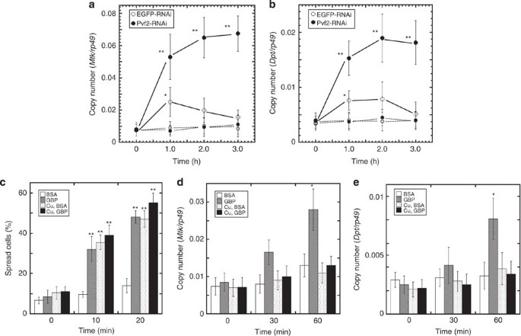Figure 5: Effects of Pvf/Pvr signalling on cellular and humoral immune responses ofDrosophilaS2 cells. (a) Effect of dsRNA targeting ofPvf2on GBP-inducedMtkexpression. Fifty nM GBP was added into each well containing 1 × 106S2 cells. Control values without GBP were shown by dotted lines. Each value represents the mean±s.d. for five independent determinations. *P<0.05; **P<0.01: Significant differences from control (0 min) value are indicated by Tukey’s HSD. (b) Effect of dsRNA targeting ofPvf2on GBP-inducedDptexpression. Other explanations are as ina. (c) Effect ofPvf2overexpression on GBP-induced S2 cell spreading.Pvf2expression was induced by addition of CuSO4into the culture medium. Fifty nM GBP or BSA was added to S2 cells for the indicated times. Each value represents the mean±s.d. for five independent determinations. **P<0.01: Significant differences from control (0 min, BSA) value are indicated by Tukey’s HSD. (d) Effect ofPvf2overexpression on GBP-inducedMtkexpression in S2 cells measured as described in (a). Each value represents the mean±s.d. for five independent determinations. *P<0.05: Significant difference from control (0 min, BSA) value is indicated by Tukey’s HSD. Other explanations are as inc. (e) Effect ofPvf2overexpression on GBP-inducedDptexpression in S2 cells measured as described inb. Other explanations are as ind. Figure 5: Effects of Pvf/Pvr signalling on cellular and humoral immune responses of Drosophila S2 cells. ( a ) Effect of dsRNA targeting of Pvf2 on GBP-induced Mtk expression. Fifty nM GBP was added into each well containing 1 × 10 6 S2 cells. Control values without GBP were shown by dotted lines. Each value represents the mean±s.d. for five independent determinations. * P <0.05; ** P <0.01: Significant differences from control (0 min) value are indicated by Tukey’s HSD. ( b ) Effect of dsRNA targeting of Pvf2 on GBP-induced Dpt expression. Other explanations are as in a . ( c ) Effect of Pvf2 overexpression on GBP-induced S2 cell spreading. Pvf2 expression was induced by addition of CuSO 4 into the culture medium. Fifty nM GBP or BSA was added to S2 cells for the indicated times. Each value represents the mean±s.d. for five independent determinations. ** P <0.01: Significant differences from control (0 min, BSA) value are indicated by Tukey’s HSD. ( d ) Effect of Pvf2 overexpression on GBP-induced Mtk expression in S2 cells measured as described in ( a ). Each value represents the mean±s.d. for five independent determinations. * P <0.05: Significant difference from control (0 min, BSA) value is indicated by Tukey’s HSD. Other explanations are as in c . ( e ) Effect of Pvf2 overexpression on GBP-induced Dpt expression in S2 cells measured as described in b . Other explanations are as in d . Full size image GBP-mediated immunopolarization in single cells Finally, we used transgenic Drosophila larvae expressing green fluorescence protein (GFP) under the control of the Mtk promoter. When we isolated plasmatocytes from the transgenic larvae injected with GBP, we found that the fluorescent signal was not uniformly distributed ( Fig. 6a ). Most of the strong fluorescent signals were found in the rounded (non-spread) plasmatocytes, but little or no signal was observed in spread cells ( Fig. 6a–c ; Supplementary Fig. 9 ). These data strongly indicated that, in the presence of GBP, a single plasmatocyte cannot simultaneously exert both arms of the immune response. We used the same reporter assay for the Mtk promoter in S2 cells ( Fig. 6d ). One hour after GBP treatment, we observed that the GFP signal was lost during the transition from non-spread to spread cells ( Fig. 6d ). We further conclude that, through its actions on individual cells, GBP enhances one arm of the immune pathway—either the humoral or cellular response—while inhibiting the other ( Fig. 6e ). We can describe this phenomenon as immunophysiological polarization. It is initiated by GBP in cooperation with the Pvf/Pvr signalling cascade. This represents a new development in our understanding of the molecular basis by which insects mount a defense against invading pathogens. 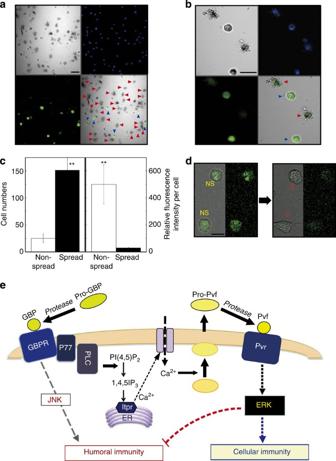Figure 6: GBP effect on a reporter assay forMetchnikowinexpression inDrosophilaplasmatocytes and S2 cells, and a model of the GBP signalling pathway. (a) Low magnification view ofDrosophilaplasmatocytes. Larvae expressingGFPunder the control of theMtkpromoter were injected with ~20 nmol per larva of GBP, 1 h before plasmatocytes were prepared. Non-spread (blue arrowhead) and spread (red arrowhead) plasmatocytes were observed by laser scanning confocal microscopy (EZ-Ti, Nikon). Scale bar, 20 μm. (b) High magnification view ofDrosophilaplasmatocytes. Other explanations are as ina. (c) Quantitative analysis of GFP expression in non-spread and spread cells. Cell morphology was scored by counting ~200 cells from a randomly selected view. Average fluorescent signal intensities of each cell were quantified by the confocal microscope software EZ-C1 (Nikon). Each value represents the mean±s.d. for four independent determinations (**P<0.01): Significant differences are indicated by Tukey’s HSD. (d) Effect of GBP on GFP expression in S2 cells expressing GFP under the control of theMtkpromoter. One hour after addition of 50 nM GBP, S2 cells were analysed by confocal microscopy as described ina. Scale bar, 10 μm. (e) Overview of the new positive and negative regulatory features of the GBP signalling pathway described in the current study: Stimulation of PLC by activated GBPR produces IP3, which promotes extracellular Ca2+influx. We have previously demonstrated the presence of GBPR together with its adaptor protein (P77) ref.38,42. Elevated Ca2+triggers secretion of Pvf which stimulates Pvr. Activation of Pvr in turn promotes ERK phosphorylation, which activates cellular immune responses (cellular immunity) such as encapsulation while simultaneously repressing the expression of immune effector molecules such as Mtk (humoral immunity). See the text for discussion of the possibility that Pvf2 may be activated by proteolysis. Figure 6: GBP effect on a reporter assay for Metchnikowin expression in Drosophila plasmatocytes and S2 cells, and a model of the GBP signalling pathway. ( a ) Low magnification view of Drosophila plasmatocytes. Larvae expressing GFP under the control of the Mtk promoter were injected with ~20 nmol per larva of GBP, 1 h before plasmatocytes were prepared. Non-spread (blue arrowhead) and spread (red arrowhead) plasmatocytes were observed by laser scanning confocal microscopy (EZ-Ti, Nikon). Scale bar, 20 μm. ( b ) High magnification view of Drosophila plasmatocytes. Other explanations are as in a . ( c ) Quantitative analysis of GFP expression in non-spread and spread cells. Cell morphology was scored by counting ~200 cells from a randomly selected view. Average fluorescent signal intensities of each cell were quantified by the confocal microscope software EZ-C1 (Nikon). Each value represents the mean±s.d. for four independent determinations (** P <0.01): Significant differences are indicated by Tukey’s HSD. ( d ) Effect of GBP on GFP expression in S2 cells expressing GFP under the control of the Mtk promoter. One hour after addition of 50 nM GBP, S2 cells were analysed by confocal microscopy as described in a . Scale bar, 10 μm. ( e ) Overview of the new positive and negative regulatory features of the GBP signalling pathway described in the current study: Stimulation of PLC by activated GBPR produces IP 3 , which promotes extracellular Ca 2+ influx. We have previously demonstrated the presence of GBPR together with its adaptor protein (P77) ref. 38 , 42 . Elevated Ca 2+ triggers secretion of Pvf which stimulates Pvr. Activation of Pvr in turn promotes ERK phosphorylation, which activates cellular immune responses (cellular immunity) such as encapsulation while simultaneously repressing the expression of immune effector molecules such as Mtk (humoral immunity). See the text for discussion of the possibility that Pvf2 may be activated by proteolysis. Full size image Our study breaks new ground by demonstrating reciprocal coordination of the humoral and cellular arms of an innate immune program in insect plasmatocytes and Drosophila S2 cells. Furthermore, we provide a molecular characterization of the signalling cascades that are responsible for this immunophysiological polarization. For example, we used the Drosophila S2 cell line to characterize a linear, multistep pathway by which GBP promotes cell spreading, a phenomenon that is generally regarded as the initiation of the cellular immune response. This work includes demonstrating a novel role in immunity for the PLC signalling system. We have further shown that the autocrine Pvf/Pvr loop is one of the signalling events that is activated downstream of GBP. This is not only a previously unknown function for GBP, but is also a finding that counters previous proposals that the Pvf/Pvr pathway is a general inhibitor of immune responses [18] , [32] . We have now demonstrated that the Pvf/Pvr pathway serves a more complex, coordinating role than was previously appreciated; its activation downstream of GBP downregulates humoral immune responses in favour of initiating a cellular-based immunity program—all in the same cells. Our characterization of GBP as a pivotal regulator of the nature of an insect’s response to invading pathogens could be pertinent to human health, since the mechanisms and principles of innate immunity are so highly conserved. The success of our study owes much to the S2 hemocyte-like cell line being a convenient, yet powerful model for studying immune responses in Drosophila [16] , [18] . While plasmatocytes can be obtained from Drosophila larvae, the isolation procedures are tedious and the yields are low. We have now added to the value of S2 cells in immunity research by demonstrating that GBP promotes spreading of these cells ( Fig. 1 ), an initial step in the acquisition of an encapsulating phenotype. The GBP provides a convenient means of determining physiological response to specific signalling activities, such the PLC/Ca 2+ cascade [16] , [23] . It was also the genetic tractability of S2 cells that allowed us to determine that Pvf knockdown strongly inhibited GBP-dependent cell spreading while upregulating expression of the humoral effector gene, Mtk . That is, the S2 cells exhibited immunopolarization. While observations made with S2 cells might not always recapitulate immunological phenomena that take place in vivo , we also observed immunopolarization in individual plasmatocytes that were obtained from Drosophila larvae treated with RNAi against Pvr : these cells exhibited enhanced expression of Mtk but impaired cell spreading ( Figs 4 and 5 ). Similar to an earlier study [8] , we found that overexpression of GBP in vivo slightly stimulated Mtk expression, but to a level that was ~10-fold less than that induced on bacterial infection ( Fig. 4d ). Previously, the significance of that observation was unclear [8] . Our current study has now clarified that the relatively weak effect of GBP overexpression in Drosophila larvae reflects a role of Pvr in downregulating humoral immune responses [18] ( Fig. 4d ). Our elucidation of these ‘gatekeeper’ roles for the Pvf/Pvr loop suggest that it may be profitable for future research to investigate whether regulation of the expression of these particular genes influences polarization of plasmatocytes between cellular and humoral phenotypes, for example, in response to the degree of the pathogenic challenge, or in response to microenvironmental fluctuations. One intriguing observation is that a few minutes treatment with the protease inhibitor APMSF led to inhibition of GBP-dependent activation of ERK via the Pvf2/Pvr signalling pathway ( Fig. 2e ). In such experiments, APMSF is not expected to enter cells [33] , [34] . Furthermore, APMSF does not affect GBP-mediated Ca 2+ mobilization ( Fig. 2c ). We therefore speculate that Pvf2 may require proteoloytic processing to be activated; that is a process that could account for sensitivity to APMSF. However, further experiments are required to investigate that possibility. It is known that innate immune responses exhibit a high degree of evolutionary conservation. For example, the platelet-derived growth factor receptor is a mammalian homologue of Drosophila Pvr [29] . Moreover, professional phagocytes in mammals—such as macrophages—undergo immunophysiological polarization [35] . This can manifest itself as a balance between competing pro- and anti-inflammatory phenotypes, and there are also instances where cellular and humoral responses are differentially regulated. The degree of polarization reflects both the nature of the threat to the host, and changes in microenvironmental conditions; the signalling mechanisms that underlie these complex responses are poorly understood [36] . Thus, the possibility that there may be a human homologue of GBP and conservation of its mechanisms of action, are both subjects that deserve further investigation. It is well recognized that innate immunity in insects involves both humoral and cellular defense strategies. These two processes are often viewed as being cooperative and functionally equivalent [3] , [11] . However, in recent years, a competing viewpoint has emerged that depicts cellular activities such as phagocytosis and encapsulation as being somewhat independent ‘first responders’ [9] , [37] . This hypothesis further depicts the induction of humoral responses, such as the transcription of AMP gene products, as a secondary, delayed response [9] , [37] . Our study provides strong new support for the latter ideas. Moreover, we show that the delay before humoral genes are induced need not be passive; that is another key conclusion to emerge from our study, which demonstrates that GBP actively restrains humoral response processes through the Pvf/Pvr signalling pathway. Further studies aimed at revealing the regulatory mechanism of Pvf/Pvr signalling activities in immune cells should enhance understanding of the overall regulation of GBP-induced immunophysiological polarization in insects. Some beneficial outcomes of this measured, GBP-dependent sequential defense strategy may be proposed. First, it is strikingly efficient to deploy a single upstream mediator—GBP—rather than a range of cross-regulatory agonists, to reciprocally regulate two different physiological responses. Second, limiting the role of the humoral defenses may minimize the negative consequences of antagonistic pleiotropy: humoral immune genes have other functions in growth and development, and so organismal homeostasis may be less perturbed while the insect attempts to first neutralize an invading pathogen by phagocytosis and encapsulation. Third, since heightened immunity has a negative impact on other life traits, a calibrated immune response may more efficiently manage the investment in resources that are required to fight infection. Our conclusion that GBP can enforce the timing of the induction of these different components of the overall immune response reveals the importance of this peptide in managing survival of the organism with minimal cost to its overall fitness. Animals and Cells P. separata larvae were reared on an artificial diet (10% kidney beans, 10% wheat bran, 4.2% dried yeast, 0.5% ascorbic acid, 0.3% antiseptic reagents and 1.3% agar) at 25 °C with a photoperiod of 16 h light: 8 h dark [38] . Drosophila melanogaster stocks were reared on cornmeal–glucose–yeast medium at 23 °C [39] . The UAS-dsPvr strains were supplied by NIG-FLY (National Institute of Genetics). The Mtk-GFP strain was gift from Jean-Luc Imler (Institut de Biologie Moléculaire et Cellulaire, Strasbourg, France) [40] . We generated Pvr knockeddown and GBP overexpressed transgenic flies controlled by the hs-Gal4 driver [8] , [41] . Drosophila S2 cells were maintained Schneider’s Drosophila medium (Gibco, USA) was supplemented with 5% fetal bovine serum (FBS), 50 units ml −1 penicillin and 50 μg ml −1 streptomycin at 25 °C. Peptides P. separata GBP (ENFSGGCVAGYMRTPDGRCKPTF), D. melanogaster GBP (ILLETTQKCKPGFELFGKRCRKPA) and Pvf2 peptide fragment (CPRPGLPNRNPNLQQRLQSKRQNGKS) were synthesized and purified by reversed-phase C 8 HPLC column (5-μm particle size, 4.6 × 250 mm, pore size=300 Å; YMC, Japan) [42] . Cell-Spreading Assay P. separata haemolymph was collected into an ice-cold microcentrifuge tube containing 1 ml of anticoagulant buffer (41 mM citric acid, 98 mM NaOH, 186 mM NaCl, 1.7 mM EDTA, pH 4.5) and immediately centrifuged at 500 g for 1 min at 4 °C. Precipitated hemocytes were suspended in 1 ml anticoagulant buffer and, after leaving on ice for 30 min, cells were used for preparation of plasmatocytes. For isolation of plasmatocytes (over 90% purity), Percoll step-gradient centrifugation was used according to the method of Clark et al . [12] Whole isolated plasmatocytes were washed twice with anticoagulant buffer and once with Ex-Cell 420 medium (JHR Bioscience, Hampshire, UK) by repeating suspending and centrifugation at 500 g . Washed cells were finally resuspended in Ex-Cell 420 medium (2 × 10 4 cells ml −1 ) containing GBP at 25 °C. The percentage of plasmatocytes spread in an assay was scored 20–30 min after mixing cells and peptide by counting 100 cells from a randomly selected view. The proportion of flattened and spread plasmatocytes was then recorded. Drosophila larval hemocytes were collected into an ice-cold microcentrifuge tube containing 100 μl of anticoagulant buffer and immediately centrifuged at 500 g for 2 min at 4 °C. Precipitated hemocytes were suspended in Schneider’s Drosophila medium (1 × 10 4 cells ml −1 ) and directly used for spreading assay, because it is known that most of the larval hemocytes (over 90%) are plasmatocytes in healthy larvae. S2 cells were collected from a stock culture flask 2–3days after seeding, and washed twice with Schneider’s Drosophila medium. Washed cells were suspended in 500 μl same medium (1 × 10 5 cells ml −1 ) and, after leaving on ice for 60 min, cells were used for spreading assays. The degree to which the normally spherical plasmatocytes (or S2 cells) adopted a more flattened, spread phenotype was assessed by micrometric analysis. Cells were regarded as spread when they became flattened with their longest axis ≥35 μm (for P. separata plasmatocytes), ≥24 μm (for D. melanogaster plasmatocytes) and ≥25 μm for (S2 cells). Quantitative RT–PCR Analysis To quantify Drosophila gene expression in Drosophila S2 cells or larval hemocytes, RT–PCR was conducted essentially according to the previously described procedure as follows [24] . Total RNAs of S2 cells or Drosophila hemocytes were prepared from larvae injected with ~20 nmol per larva GBP or BSA 60 min after the injection. First-strand cDNA was synthesized with oligo(dT) 12−18 primer using ReverTra Ace RT–PCR kit (Toyobo, Japan) according to the manufacturer’s protocol. The cDNAs for target genes were amplified with a specific primer pair indicated in Supplementary Table 1 . PCR was conducted under the following conditions: 20–28 cycles at 95 °C for 30 s, 58 °C for 30 s, and 72 °C for 45 s. Quantitative real-time PCR was carried out with the cDNAs in a 20 μl reaction volume of LightCycler Fast DNA Master SYBR Green I (Roche Applied Science, USA), using the Light-Cycler 1.2 instrument and software (Roche Applied Science). The PCR cycling conditions were denaturation at 95 °C for 10 min, followed by 45 cycles of 95 °C for 10 s, annealing at 55 °C for 5 s and extension at 72 °C for 15 s. Using the second derivative maximum method provided in the LightCycler software (version 3.5), a standard curve was generated by plotting the external standard concentration against threshold cycle. The software automatically calculated PCR product concentration for each tissue sample. All samples were analysed in duplicate, and assay variation was typically within 10%. Data were normalized according to the expression level of rp49 determined in duplicate by reference to a serial dilution calibration curve. All primers used in this study were listed in Supplementary Table 1 . Measurements of inositol phosphates All experiments were performed at 25 °C. S2 cells (6-well dish; each well contained 5 × 10 5 cells in 2 ml) were labelled for 4 days with [ 3 H] myo -inositol (Perkin Elmer; 35 μCi per ml). After 2 days, fresh media and [ 3 H] myo -inositol were added. On day 4, the medium was replaced with a serum-free medium (either Schneider’s Drosophila medium or HEPES-buffered salt solution (120 mM NaCl, 20 mM HEPES (pH 7.4 with NaOH), 5.4 mM KCl, 0.8 mM MgCl 2 , 10 mM glucose, and unless otherwise stated, 1 mM CaCl 2 ). After a further 1–3 h, LiCl was added to a final concentration of 10 mM for 20 min and then Drosophila GBP was added for various times. Assays were quenched by aspiration of media followed immediately by the addition of 1 ml ice-cold 0.6 M perchloric acid per 0.02 mM InsP 6 . After 20 min on ice, soluble material was removed and neutralized with 0.4 ml of 1 M potassium bicarbonate/0.04 M EDTA. Samples were stored at 4 °C overnight, centrifuged to remove insoluble potassium perchlorate, diluted 1:1 with 1 mM EDTA and then analysed either by a Q-100 HPLC (4.6 × 250 mm; Thomson Instruments, USA) with an in-line detector [23] . Double-stranded RNA-mediated interference in vitro Individual DNA fragments ~700 bp in length, containing coding sequences for the proteins to be ‘knocked down’ were amplified by using PCR. Each primer used in the PCR contained a 5′ T7 RNA polymerase binding site (5′- GAATTAATACGACTCACTATAGGGAGA -3′) followed by sequences specific for the targeted genes (see Supplementary Table 1 ). The PCR products were purified and were used as templates by using a Megascript T7 transcription Kit (Ambion, USA) to produce dsRNA according to the manufacturer’s protocol. Ten micrograms of dsRNA were analysed by 1.5% agarose gel electrophoresis to ensure that the majority of the dsRNA existed as a single band of ~700 bp. S2 cells were incubated at 1 × 10 5 cells per well in 96-well plate in 1 × Schneider’s Drosophila media with 5% FBS at 25 °C. dsRNA was added directly to the media to a final concentration of 37 nM. The cells were incubated for three days to allow for turnover of the target protein. Expression of Pvf2 or Mtk-GFP in Drosophila S2 cells Overexpression of Pvf2 in Drosophila S2 cells were performed using pCoHygro vector (Invitrogen) according to procedure of Kellenberger et al . [43] Cells were used 3–4 days following induction of Pvf2 by addition of 0.5 mM CuSO 4 , S2 cells were used for a series of assays. The Mtk-GFP construct (1,495 bp of Mtk upstream sequences fused with the jellyfish Aequorea victoria GFP ) [40] was cloned into the pMT-V5 His vector and co-transfected into S2 cells with pCoHygro vector. S2 cells were propagated in 1 × Schneider’s Drosophila medium with 5% FBS at 25 °C. Analysis of ERK phosphorylation S2 cells were collected into an ice-cold microcentrifuge tube containing 1 ml of anticoagulant buffer and immediately washed twice with anticoagulant buffer. Washed cells were solubilized by adding same volume of 2 × lysis buffer (100 mM HEPES-NaOH, 300 mM NaCl, 3 mM MgCl 2 , 1 mM EDTA, 20% glycerol, 2% TX-100 (w/v), 1% sodium deoxycholate, 0.2% SDS, pH 7.5) containing Protease inhibitor cocktail (Nacalai tesque, Japan), phosphatase inhibitor cocktail set II (Calbiochem, USA), and 0.2% phenylthiourea. After centrifugation at 17,000 g for 15 min at 4 °C, the supernatant was mixed with the same volume of sample buffer (125 mM Tris–HCl, 10% 2-mercaptoethanol, 4% SDS, 10% sucrose, 0.004% bromophenol blue) and separated by SDS–PAGE (8 or 10%), transferred onto an Immobilon-P PVDF membrane (Millipore, USA). Proteins on the membrane were probed with anti-activated MAP Kinase (diphosphorylated ERK-1&2) mouse monoclonal antibodies (at 1:2,000, M9692, Sigma-Aldrich, USA) [38] . For reprobing, membranes were washed for 30 min at 50 °C in 62.5 mM Tris–HCl (pH 6.7) containing 100 mM 2-mercaptoethanol and 2% SDS, and they were probed with anti-MAP kinase (ERK-1&2) mouse monoclonal antibodies (at 1:2,000, M5670, Sigma-Aldrich, USA). All positive bands were quantified using ImageJ (NIH). Immunoblotting of Pvf2 The carboxy-terminal 26-amino-acid peptide of Pvf2 was coupled to keyhole limpet haemocyanin using the carbodiimide cross-linker, 1-ethyl-3-(3-dimethylaminopropyl)carbodiimide hydrochloride, emulsified in Titer Max Gold (CytRx, USA) and subcutaneously injected into a female rabbit to generate a specific polyclonal antibody. Anti-Pvf2 IgG was precipitated by adding ammonium sulphate to 40% saturation and further purified by an affinity column of protein G-Sepharose (GE Healthcare, USA). After collecting S2 culture medium, the medium was immediately mixed with −20 °C acetonitrile (final 30%) and centrifuged at 20,000 g . for 10 min at 4 °C. The supernatant was concentrated by lyophilization, separated by SDS/PAGE and electrically transferred to a PVDF membrane filter. After blocking with BSA, polypeptides on the membrane were probed with anti-Pvf2 antibody (at 1:1,000) [38] . Measurements of Ca 2+ response using GCaMP3-expressing Drosophila S2 S2 cell line that stably expresses GCaMP3 was established by co-transfection with pCoBlast and GCaMP3 harbouring pAc5.1/V5-HisA vectors using a Calcium Phosphate Transfection Kit basically according to the manufacture’s instruction (Invitrogen, USA). GCaMP3-expressing S2 cells were collected from a stock culture flask 3–4 days after seeding, and washed twice washed twice and incubated in Schneider’s yeast-extract free and serum-free Drosophila medium (US Biological, USA). Approximately 1 × 10 5 cells per well were plated in 96-well plates and incubated for 1 h at 25 °C in 200 μl medium, before the addition of indicated test samples. Calcium-induced fluorescence changes were recorded simultaneously in all wells using a FLIPR-TETRA (Molecular Devices). Analysis of GFP expression in plasmatocytes and Drosophila S2 cells Whole haemolymph was collected from Drosophila larvae expressing Mtk-GFP into a 20 μl drop of chilled Schneider’s Drosophila medium (Invitrogen) 1 h after injection of ~0.10 μl of 200 mM GBP. Soon after collecting haemolymph from 10 larvae, hemocytes were sedimented by centrifugation at 4 °C for 2 min at 500 g and suspended in Schneider’s Drosophila medium. After nuclear staining with Hoechst 33258, fluorescence of GFP in hemocytes was monitored by laser scanning confocal microscope (EZ-Ti system, Nikon) using a 488-nm excitation filter in combination with a 515-nm emission filter. S2 cells were also observed in the same way by the confocal microscope. To quantify fluorescent intensities in each cell, we analysed approximately 200 cells from a randomly selected view and identified as non-spread and spread cells by micrometric analysis. We next measured fluorescent intensities in these cells by the confocal software EZ-C1 (Nikon) and these values were divided by the cell areas. We performed this analysis for control and GBP-treated cells. Infection and injury experiments Direct bacterial infection experiments was induced by stabbing third instar larvae with a thin tungsten needle (diameter: ~0.05 mm) previously dipped into a concentrated culture of Serratia marcescens (OD 600 =1 × 10 −2 ). Statistics Statistical significance was examined by analysis of variance with a Tukey’s HSD post hoc test. How to cite this article : Tsuzuki, S. et al . Switching between humoral and cellular immune responses in Drosophila is guided by the cytokine GBP. Nat. Commun. 5:4628 doi: 10.1038/ncomms5628 (2014).